Engineering transkingdom signalling in plants to control gene expression in rhizosphere bacteria 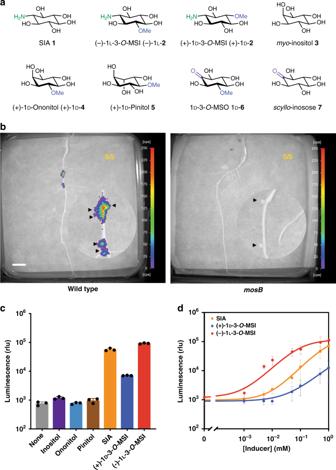Fig. 1 Detection of rhizopine exudation with a rhizopine biosensor.aChemical structures of rhizopines and related cyclitols.bNightOwl images of bioluminescence ofR. leguminosarumRlv3841/pOPS0046 rhizopineluxbiosensor on the surface ofM. sativaroots nodulated byS. melilotiL5-30 wild-type (rhizopine+) andS. melilotiL5-30mosB:pK19 (rhizopine –, see Fig.2a). Numbers in top right corners indicate number of plants tested that showed significant levels of bioluminescence (n= 5). Circle in bottom right corner contains magnified image of a root section enriched with nodules. The positions of nodules are indicated with arrowheads (scale bar, 1 cm). Colours represent luminescence intensity from 0 counts per second (cool/purple) to 250 counts per second (warm/red).cSpecificity of induction of rhizopineluxbiosensor with rhizopines compared to other chemically similar plant polyols, grown in UMS minimal medium with pyruvate and ammonia as carbon and nitrogen sources, supplemented with 1 mM of inducing molecule. Data are presented as relative luminescence units (rlu). Black dots indicate individual data points for each condition.dInduction curves showing the dynamic range and sensitivity of the rhizopineluxbiosensor with chemically synthesised SIA1, (−)-1l-3-O-MSI (−)-1l-2and (+)-1d-3-O-MSI (+)-1d-2grown in UMS minimal medium with pyruvate and ammonia as carbon and nitrogen sources. Error bars represent standard deviation of the mean ofn= 3 independent replicates. All experiments were repeated at least three independent times The root microbiota is critical for agricultural yield, with growth-promoting bacteria able to solubilise phosphate, produce plant growth hormones, antagonise pathogens and fix N 2 . Plants control the microorganisms in their immediate environment and this is at least in part through direct selection, the immune system, and interactions with other microorganisms. Considering the importance of the root microbiota for crop yields it is attractive to artificially regulate this environment to optimise agricultural productivity. Towards this aim we express a synthetic pathway for the production of the rhizopine scyllo -inosamine in plants. We demonstrate the production of this bacterial derived signal in both Medicago truncatula and barley and show its perception by rhizosphere bacteria, containing bioluminescent and fluorescent biosensors. This study lays the groundwork for synthetic signalling networks between plants and bacteria, allowing the targeted regulation of bacterial gene expression in the rhizosphere for delivery of useful functions to plants. The root microbiota, like the gut microbiota in human health, is critical for plant health and agricultural yield [1] , [2] . It is shaped by plant selection [3] , [4] and its immune system [5] , as well as complex interactions between microorganisms. Plant growth-promoting bacteria can alter nutrient availability and antagonise pathogens. Perhaps, the most important plant–microbe interaction is between legume plants and symbiotic bacteria called rhizobia. Natural transkingdom signalling between them is essential for the establishment of rhizobia in plant root organs called nodules. In root nodules rhizobia reduce atmospheric N 2 to ammonia, producing a substantial proportion of the biosphere’s available nitrogen. The root microbiota represents an enormous potential for improving crop yields by engineering the plant microbiome. Enhancing crop productivity in a sustainable manner may be achieved in several ways, including transfer of bacterial N 2 fixation to cereals [6] , [7] , [8] , [9] , harnessing bacterial phosphate solubilisation, promoting root growth by bacterial synthesis of plant hormones, or pathogen antagonism by antibiotic production. These plant growth-promoting services by bacteria could be regulated by engineering plants to produce a synthetic transkingdom signal to control bacteria on roots. Such a signal must be: (1) amenable to engineering in plants, (2) able to elicit a bacterial response, (3) exuded into the rhizosphere (zone of soil surrounding the roots) and (4) not normally be made by plants. Transgenic plants that produced opine molecules, repurposed from Agrobacterium , have been shown to enrich their rhizosphere with bacteria able to catabolize opines; however, utilizing a nutritional mediator of pathogenic organisms as a signal is undesirable [10] , [11] , [12] . A group of compounds, called rhizopines, were recognised as ideal chemical signals, although efforts to engineer rhizopine-producing plants in the past were unsuccessful [13] . Rhizopines ( scyllo -inosamine 1 (SIA) and 3- O -methyl- scyllo -inosamine 2 (3 -O -MSI)) (Fig. 1a ) are synthesised by a few species of rhizobia in legume nodules, under the control of the NifA regulator, during N 2 -fixing symbiosis [14] . These molecules are rare in nature [15] and absent from most plant rhizospheres. Rhizobia are able to synthesise rhizopines and utilise them as carbon and nitrogen sources. Genes involved in the biosynthesis ( mosABC ) and catabolism of rhizopines ( mocCABRDEF ) have been identified in the wild-type rhizobium Sinorhizobium meliloti L5-30 [16] , [17] . Although the natural role of rhizopines remains to be elucidated, previous studies suggested that they may be exuded into the rhizosphere [14] , [18] . Fig. 1 Detection of rhizopine exudation with a rhizopine biosensor. a Chemical structures of rhizopines and related cyclitols. b NightOwl images of bioluminescence of R. leguminosarum Rlv3841/pOPS0046 rhizopine lux biosensor on the surface of M. sativa roots nodulated by S. meliloti L5-30 wild-type (rhizopine+) and S. meliloti L5-30 mosB :pK19 (rhizopine –, see Fig. 2a ). Numbers in top right corners indicate number of plants tested that showed significant levels of bioluminescence ( n = 5). Circle in bottom right corner contains magnified image of a root section enriched with nodules. The positions of nodules are indicated with arrowheads (scale bar, 1 cm). Colours represent luminescence intensity from 0 counts per second (cool/purple) to 250 counts per second (warm/red). c Specificity of induction of rhizopine lux biosensor with rhizopines compared to other chemically similar plant polyols, grown in UMS minimal medium with pyruvate and ammonia as carbon and nitrogen sources, supplemented with 1 mM of inducing molecule. Data are presented as relative luminescence units (rlu). Black dots indicate individual data points for each condition. d Induction curves showing the dynamic range and sensitivity of the rhizopine lux biosensor with chemically synthesised SIA 1 , (−)-1 l -3- O -MSI (−)-1 l - 2 and (+)-1 d -3- O -MSI (+)-1 d - 2 grown in UMS minimal medium with pyruvate and ammonia as carbon and nitrogen sources. Error bars represent standard deviation of the mean of n = 3 independent replicates. All experiments were repeated at least three independent times Full size image In this study, we demonstrate the exudation of rhizopines into the rhizosphere by a rhizobium–legume symbiosis and elucidate the biochemical pathway for 3- O -MSI 2 biosynthesis by rhizobia in legume nodules. We show that while the 3- O -MSI 2 biosynthetic pathway is not readily amenable to transfer to plants, the biosynthesis of the rhizopine SIA 1 is. Finally, we establish synthetic SIA-mediated transkingdom signalling from transgenic Medicago truncatula and barley plants to bacteria in their rhizospheres. Rhizopine exudation during rhizobial symbiosis To validate rhizopines as targets for transkingdom signalling, we first wished to confirm they are exuded into the plant rhizosphere in their natural context (synthesis by rhizobia in N 2 -fixing root nodules). To investigate exudation into the rhizosphere, a rhizopine biosensor (pOPS0046) was made by cloning the mocB promoter (encodes a putative ATP transporter substrate-binding protein in the rhizopine catabolism locus) and its divergent regulator mocR [19] into a lux reporter vector [20] . Exudation of rhizopine into the rhizosphere was measured by bacterial luminescence on roots [20] of the natural host of S. meliloti L5-30, Medicago sativa . Plants were co-inoculated with S. meliloti L5-30 (which nodulates and produces rhizopine) and Rhizobium leguminosarum (Rlv3841) carrying pOPS0046 (contains the biosensor but cannot nodulate). Medicago sativa plants nodulated by S. meliloti L5-30 caused bioreporter Rlv3841 to bioluminesce on the root surface adjacent to nodules (Fig. 1b , Supplementary Fig. 1 ), confirming rhizopines traverse plant tissues to reach the root surface. To confirm that the biosensor responds specifically to rhizopines, SIA 1 was obtained via a revised synthetic route, and both enantiomers of 3- O- MSI, (−)-1 l - 2 and (+)-1 d - 2 , were synthesised using a protection-resolution strategy (Supplementary Figs. 2 and 3 ). The absolute configuration of key synthetic intermediates was confirmed by nuclear magnetic resonance analysis (Supplementary Table 5 ) and single-crystal X-ray diffraction. Induction of the biosensor was tested in free-living culture in response to SIA 1 , (−)-1 l -3- O -MSI (−)-1 l - 2 and (+)-1 d -3- O -MSI (+)-1 d - 2 , and the naturally abundant cyclitols myo -inositol 3 , ( + ) -1d- ononitol ( + )-1d- 4 and ( + )-1d- pinitol ( + )-1d - 5 (Fig. 1a ). The biosensor was activated by SIA 1 and (−)-1 l -3- O -MSI (−)-1 l - 2 (Fig. 1c, d ). (−)-1 l -3- O -MSI (−)-1 l - 2 has previously been proposed to be the naturally occurring enantiomer [21] , and the preference for this enantiomer observed in Fig. 1c, d supports this. Furthermore, (−)-1 l -3- O -MSI (−)-1 l - 2 promoted the growth of S. meliloti L5-30, whereas (+)-1 d -3- O -MSI ( + )-1d- 2 did not (Supplementary Fig. 4 ), supporting results from a recent study [21] . The confirmation of the chemical structure of rhizopines, and their secretion into the rhizosphere, provides a unique opportunity to use them as target molecules for engineering plant control of root bacteria. Elucidation of the natural 3- O -MSI biosynthetic pathway In S. meliloti L5-30 the genes mosABC were proposed to encode the pathway for 3- O -MSI biosynthesis [13] , [17] . MosA was thought to be a methyltransferase [22] , while MosB and MosC are homologous to aminotransferase and transmembrane transport proteins, respectively [13] , [16] . However, rhizopines were not produced when mosABC was expressed in Arabidopsis thaliana [13] . Furthermore, the role of MosA in 3- O -MSI synthesis has been questioned [23] , suggesting mosABC may not encode the complete rhizopine pathway. Bioinformatic analysis of rhizobial genomes indicated that mosA is not widely distributed among putative rhizopine loci (Supplementary Fig. 5 ). 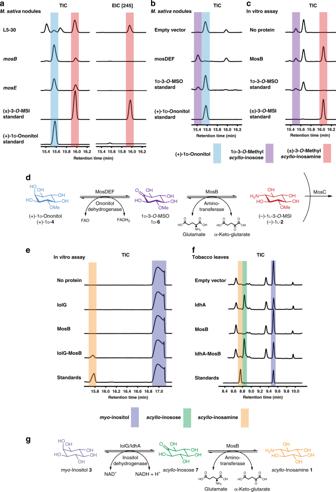Fig. 2 Discovery of a natural and synthetic pathway for rhizopine synthesis.aGas chromatography-mass spectrometry (GC-MS) total ion chromatograms (TICs) (left) and extracted ion chromatograms (m/z245 = 3-O-MSI-TMS) (EIC [245]) (right) of metabolites from nodules formed by wild-typeS. melilotiL5-30 compared tomosB:pK19 andmosE:pK19 mutants. Chemically synthesised (±)-3-O-MSI (±)-2and purchased (+)-1d-ononitol (+)-1d-4as standards are shown below.bGC-MS chromatograms of metabolites from nodules formed by wild-typeS. melilotiRm1021 maintaining an empty vector (EV) and expressingmosDEF. Chemically synthesised (±)-3-O-methyl-scyllo-inosose (±)-6and purchased (+)-1d-ononitol (+)-1d-4as standards are shown below.cGC-MS chromatograms (TIC) of MosB in vitro assay in the absence of protein or with MosB added. Chemically synthesised (±)-3-O-methyl-scyllo-inosose (±)-6and (±)-3-O-MSI (±)-2 as standards are shown below.dProposed natural pathway of 3-O-MSI biosynthesis inS. melilotiL5-30.eLinked in vitro assay of inositol dehydrogenase IolG and MosB. GC-MS TICs of assay mix in the absence of added protein, with IolG added, with MosB added and with IolG and MosB added together. Standards represent a mix of SIA1andmyo-inositol3.fGC-MS TICs of extracts prepared from tobacco leaves agro-infiltrated with either empty vector (control) or IdhA or MosB or IdhA-MosB together. Standards represent a mix of SIA1andmyo-inositol3.gProposed synthetic pathway of SIA1synthesis. Metabolites were identified by comparison with authentic standards. Highlighted peaks indicatescyllo-inosamine1(orange),scyllo-inosose7(green),myo-inositol3(dark blue), (+)-1d-ononitol4(light blue), 1d-3-O-methyl-scyllo-inosose6(purple) and (−)-1l-3-O-methyl-scyllo-inosamine2(3-O-MSI) (red). All chromatograms are representative of experiments repeated at least three independent times. Source data underlyinga–c,eandfare provided as aSource Datafile In addition, three genes, which we name mosDEF , were found downstream of mosC in many putative rhizopine loci. Comparative analytical chemistry by gas chromatography-mass spectrometry (GC-MS), using nodule extracts from several of these rhizobia and chemically synthesised (±)-3- O -MSI (±)- 2 as a standard, revealed that mosBCDEF are present in all rhizobia that synthesised 3- O -MSI (Supplementary Fig. 5 ). Supporting the role of mosDEF in 3- O -MSI synthesis, a S. meliloti L5-30 strain disrupted in mosE showed no detectable rhizopine synthesis in nodules (Fig. 2a ). Based on homology, MosDEF is likely to be a membrane-bound flavin adenine dinucleotide-dependent dehydrogenase complex [24] . We hypothesized that the dehydrogenase complex, MosDEF, oxidises ( + )-1d- ononitol ( + )-1d- 4 at the axial C-2 hydroxyl group to form 3- O -methyl- scyllo -inosose 1d- 6 . This keto-inositol intermediate could undergo reductive amination catalysed by MosB to generate (−)-1 l- 3- O -MSI (−)-1 l- 2 . Fig. 2 Discovery of a natural and synthetic pathway for rhizopine synthesis. a Gas chromatography-mass spectrometry (GC-MS) total ion chromatograms (TICs) (left) and extracted ion chromatograms ( m/z 245 = 3- O -MSI-TMS) (EIC [245]) (right) of metabolites from nodules formed by wild-type S. meliloti L5-30 compared to mosB :pK19 and mosE :pK19 mutants. Chemically synthesised (±)-3- O -MSI (±)- 2 and purchased (+)-1 d -ononitol (+)-1 d - 4 as standards are shown below. b GC-MS chromatograms of metabolites from nodules formed by wild-type S. meliloti Rm1021 maintaining an empty vector (EV) and expressing mosDEF . Chemically synthesised (±)-3- O- methyl- scyllo -inosose (±)- 6 and purchased (+)-1 d -ononitol (+)-1 d - 4 as standards are shown below. c GC-MS chromatograms (TIC) of MosB in vitro assay in the absence of protein or with MosB added. Chemically synthesised (±)-3- O- methyl- scyllo -inosose (±)- 6 and (±)-3- O -MSI (±)-2 as standards are shown below. d Proposed natural pathway of 3- O- MSI biosynthesis in S. meliloti L5-30. e Linked in vitro assay of inositol dehydrogenase IolG and MosB. GC-MS TICs of assay mix in the absence of added protein, with IolG added, with MosB added and with IolG and MosB added together. Standards represent a mix of SIA 1 and myo -inositol 3 . f GC-MS TICs of extracts prepared from tobacco leaves agro-infiltrated with either empty vector (control) or IdhA or MosB or IdhA-MosB together. Standards represent a mix of SIA 1 and myo -inositol 3 . g Proposed synthetic pathway of SIA 1 synthesis. Metabolites were identified by comparison with authentic standards. Highlighted peaks indicate scyllo -inosamine 1 (orange), scyllo -inosose 7 (green), myo -inositol 3 (dark blue), (+)-1 d -ononitol 4 (light blue), 1 d - 3 - O -methyl- scyllo -inosose 6 (purple) and (−)-1 l -3- O -methyl- scyllo -inosamine 2 (3- O -MSI) (red). All chromatograms are representative of experiments repeated at least three independent times. Source data underlying a – c , e and f are provided as a Source Data file Full size image To test this hypothesis, mosDEF was expressed in S. meliloti Rm1021 nodules (strain that does not produce rhizopines) and a compound accumulated that had an identical retention time and mass spectrum to a peak that eluted immediately before ( + )-1d- ononitol ( + )-1d- 4 in nodules produced by wild-type S. meliloti L5-30, but not in mosE or mosB mutants (Fig. 2a, b ). We hypothesized that this compound was 3- O -methyl- scyllo- inosose 6 . To identify this compound, (±)-3- O -methyl- scyllo- inosose (±)- 6 was synthesised to serve as a chemical standard in GC-MS experiments. Although chemically synthesised (±)-3- O -methyl- scyllo- inosose (±)- 6 was unstable in solution, following derivatisation and GC-MS analysis, a unique peak was observed with an identical retention time and mass spectrum to the compound produced in nodules formed by Rm1021 expressing mosDEF (Fig. 2b ). This result is consistent with MosDEF being an ononitol dehydrogenase. Neither mosE nor mosB mutants appeared to accumulate (±)-3- O -methyl- scyllo- inosose (±)- 6 , but both accumulated substantial amounts of ( + )-1d- ononitol ( + )-1d- 4 (Fig. 2a ). The absence of accumulation of (±)-3- O -methyl- scyllo- inosose (±)- 6 in mosE is predictable. However, its absence in mosB may be caused by spontaneous conversion to ( + )-1d- ononitol ( + )-1d- 4 , as observed in our chemical standard, or due to polarity of the mosB insertion mutation on mosDEF transcription. Next, MosB was purified and when incubated with chemically synthesised 3- O -methyl- scyllo- inosose (±)- 6 , the cofactor pyridoxal 5′-phosphate (PLP), and l -glutamate, 3- O -MSI 2 was produced (Fig. 2c , Supplementary Fig. 6a ). Therefore, MosB functions as a 3- O -methyl- scyllo- inosose: l -glutamate aminotransferase generating 3- O -MSI 2 . Initial tests of 3- O -MSI synthesis in plants using Agrobacterium -mediated transient expression of McIMT (encodes myo -inositol O -methyltransferase to produce ( + )-1d- ononitol ( + )-1d- 4 from myo- inositol 3 ), mosDEF and mosB together in Nicotiana benthamiana leaves did not yield 3- O -MSI 2 (Supplementary Fig. 7 ). MosDEF may need to interact with the bacterial membrane and/or the symbiotic bacterial electron transport chain to oxidise ( + )-1d- ononitol ( + )-1d- 4 to 1d- 3- O -methyl- scyllo- inosose 1d- 6 (the substrate for MosB). Engineering of SI biosynthesis in plants To date, MosDEF is the only ( + )-1d- ononitol dehydrogenase identified, making transfer of the natural pathway of 3- O -MSI synthesis to plants difficult; therefore, an alternative was sought. Since MosB uses 3- O -methyl- scyllo- inosose 6 as the substrate backbone for transamination by l -glutamate, we considered that scyllo -inosose 7 (produced from myo -inositol 3 by bacterial inositol dehydrogenase [25] , [26] ) may also act as a transamination substrate for MosB to generate SIA 1 . IolG, the myo -inositol dehydrogenase from the Gram-positive bacterium Bacillus subtilis has been crystallized and the subject of extensive biochemical characterization [27] , [28] , [29] , [30] , and we previously identified a myo- inositol dehydrogenase in the Gram-negative R. leguminosarum (IdhA) [26] . We tested both myo- inositol dehydrogenases for activity in plants and similar activity was observed for both iolG and idhA in N. benthamiana after transient infection (Supplementary Fig. 8 ). Following protein purification B. subtilis inositol dehydrogenase (IolG) showed higher activity in vitro (Supplementary Fig. 9 ), and was used in an in vitro assay of MosB scyllo -inosose: l -glutamate aminotransferase activity. While IolG showed robust enzyme activity in vitro, we were unable to observe scyllo -inosose 7 accumulation by GC-MS. We expect this was a result of instability of scyllo -inosose 7 in aqueous solutions, which we observed when we attempted its chemical synthesis. Nevertheless, when IolG was combined with MosB, myo- inositol 3 and NAD + (substrate/cofactor for IolG), as well as l -glutamate and PLP, SIA 1 was only produced in the presence of both IolG and MosB (Fig. 2e , Supplementary Fig. 6b ). Therefore, MosB also has scyllo -inosose: l -glutamate aminotransferase activity to generate SIA 1 . In this synthetic pathway, bacterial inositol dehydrogenase oxidises myo- inositol 3 to scyllo -inosose 7 and MosB catalyses the glutamate transamination of 7 to generate SIA 1 (Fig. 2g ). We expected this synthetic pathway to be amenable to transfer of SIA synthesis into plants. To test whether this synthetic pathway is transferable to plants, inositol dehydrogenase from R. leguminosaurum (IdhA) and scyllo -inosose: l -glutamate aminotransferase (MosB) from S. meliloti were expressed in N. benthamiana leaves, and SIA 1 was produced (Fig. 2f , Supplementary Fig. 10 ). This represents the first successful transkingdom transfer of rhizopine (SIA) synthesis from bacteria to plants. Furthermore, it should enable control of members of the plant microbiota using the MocR regulator that responds to SIA 1 (Fig. 1c ). Establishment of rhizopine transkingdom signalling To demonstrate the potential of rhizopine as a transkingdom signal to bacteria in the rhizosphere, the synthetic pathway was transferred by Agrobacterium rhizogenes -mediated root transformation into Medicago truncatula . SIA was detected in transgenic hairy roots as well as in transgenic root organ cultures of M. truncatula expressing idhA and mosB under the control of constitutive promoters (Fig. 3a , Supplementary Fig. 11 ). Medicago truncatula hairy roots were found to produce 27.39 ng mg −1 dry weight SIA [SE = 9.38; N = 3] (Supplementary Data 1 ) and SIA 1 was exuded into the rhizosphere at sufficient levels for Rlv3841, carrying the rhizopine lux biosensor, to luminesce (Fig. 3c , Supplementary Fig. 11 ). No luminescence was observed when the rhizopine lux biosensor was inoculated on the transgenic roots constitutively expressing idhA alone that produced scyllo -inosose (Supplementary Fig. 12 ). This confirmed that rhizopine acts as a transkingdom signal to bacteria, rather than the scyllo -inosose intermediate, in the rhizopine synthetic pathway engineered into plants. Fig. 3 Rhizopine biosynthesis and signalling in M. truncatula and barley roots. a , b Gas chromatography-mass spectrometry (GC-MS) total ion chromatograms (TICs) of extracts prepared from M. truncatula transgenic roots ( a ) and transgenic T 0 barley seedlings ( b ) transformed with empty vector (control) or IdhA-MosB together. Highlighted peaks indicate scyllo -inosamine 1 (orange), scyllo -inosose 7 (green) and myo -inositol 3 (dark blue). All chromatograms are representative of experiments repeated at least three independent times. Source data for GC-MS chromatograms are provided as a Source Data file in Supplementary Materials. c , d NightOwl images showing bioluminescence of Rlv3841/pOPS0046 rhizopine lux biosensor on the surface of M. truncatula transgenic roots ( c ) and T 0 barley seedlings ( d ) transformed with empty vector (control) or IdhA-MosB together (engineered). Numbers in top right corners indicate number of plants tested that showed significant levels of bioluminescence (scale bar, 1 cm). Colours represent luminescence intensity from 10 or 20 counts per second (cool/purple) to 150 counts per second (warm/red). Source data underlying a , b are provided as a Source Data file Full size image The most important targets for transfer of rhizopine-mediated transkingdom signalling are cereals, where there are large global efforts to engineer plant growth promotion, disease resistance and N 2 fixation by bacteria. To assess if we could engineer rhizopine synthesis in cereals, we transferred the rhizopine biosynthesis genes into Hordeum vulgare (barley). SIA 1 production was observed in transgenic roots of T 0 and T 1 barley plants by GC-MS analysis (Fig. 3b ). T 0 and T 1 barley plants were found to produce 6.55 ng mg −1 dry weight [SE = 0.43; n = 10] and 7.00 ng mg −1 dry weight [SE = 0.17; n = 10, N = 2] of rhizopine in their transgenic roots, respectively (Supplementary Data 2 – 4 ). SIA 1 produced in transgenic roots of T 0 barley plants acted as a transkingdom signal to bacteria containing the rhizopine lux biosensor (Fig. 3d ). As cereals are our intended final target plants and transgenic seed is available for rhizopine secreting barley, we measured the signalling between barley roots and bacteria in the rhizosphere using a green fluorescent protein (GFP) rhizopine biosensor. Confocal images revealed that rhizopine produced in transgenic roots of T 1 barley plants induced GFP fluorescence at a significant level in most bacterial colonies carrying the rhizopine GFP biosensor on the root surface (Fig. 4a, b ). Thus, a circuit of plant-dependent synthesis and signalling by SIA 1 to bacteria in the rhizosphere has been established. Fig. 4 Fluorescent microscopy of rhizopine-mediated transkingdom signalling. a Confocal fluorescence microscopy images showing green fluorescent protein (GFP) fluorescence of Rlv3841::mTn7-mCherry/pOPS0761 biosensor [with constitutive mCherry fluorescence] on the surface of T 1 barley seedlings transformed with empty vector (control) or IdhA-MosB together (engineered). Z-stack projections of green fluorescence channel (left, GFP), red fluorescence channel (middle, mCherry) and all channels merged (right, bright-field) are shown (scale bars, 100 µm). Images shown are representative of experiments repeated two independent times. b Three-dimensional images of GFP/mCherry mean intensity ratios in Rlv3841::mTn7-mCherry/pOPS0761 biosensor on the surface of T 1 barley seedlings transformed with empty vector (left, control) or IdhA-MosB together (middle, engineered) (scale bars, 100 µm). Cool colours (purple) indicate low GFP/mCherry intensity ratio, and warm colours (red) indicate a high GFP/mCherry intensity ratio. Violin plot of GFP/mCherry ratios in the biosensor colonies (right; n > 75 spots; N = 3 plants). Asterisks signify statistical significance (Wilcoxon’s signed-rank test, P = 1.30 × 10 −14 ). Images shown are representative of experiments repeated two independent times Full size image The synthetic transkingdom signalling pathway established in this work opens up the microbial pan-genome to plant control. For example, it could activate specific members of the microbiota to fix N 2 , produce antibiotics or hormones, chelate iron or solubilise soil nutrients [31] . Control of these traits by the host plant would prevent off-target effects in species such as weeds that would be caused by constitutive expression. Furthermore, the inducible expression system we established here will help alleviate growth penalties incurred by constitutive overexpression of energetically intensive plant growth promotion traits in microbes. Finally, escape of genetically modified bacterial inoculants into the environment could be addressed by integrating plant signal recognition with biocontainment strategies [32] . A key example requiring host control of a microbe is the aim of transferring N 2 fixation to alleviate the demand for chemical fertilizers in agriculture. To achieve this aim, cereals must control N 2 fixation by bacteria that grow on either the surface of roots (epiphytes), inside roots (endophytes) or by bacteria that reside in engineered nodules [7] , [8] , [9] . In analogy to natural transkingdom signalling used by legumes to control rhizobial symbioses, rhizopine transkingdom signalling could control synthetic symbioses to deliver nitrogen to cereal crops. Bacterial strains and growth media Bacterial strains and plasmids used are shown in Supplementary Tables 1 and 2 , respectively. Escherichia coli strains were grown at 37 °C in Luria–Bertani (LB) medium [33] with antibiotics: ampicillin (100 μg ml −1 ), tetracycline (10 μg ml −1 ), gentamicin (10 μg ml −1 ), or kanamycin 20 μg ml −1 ). Rhizobium leguminosarum and Sinorhizobium meliloti strains were grown in tryptone yeast (TY) medium [34] or universal minimal salts (UMS) [20] at 28 °C. Antibiotics added to TY included streptomycin (500 μg ml −1 ), tetracycline (5 μg ml −1 ) and gentamicin (20 μg ml −1 ) for R. leguminosarum , and streptomycin (200 μg ml −1 ) or neomycin (80 μg ml −1 for plasmids or 200 μg ml −1 for pK19 mutants) for S. meliloti . Agrobacterium tumefaciens and A. rhizogenes were cultured in LB medium at 28 °C with antibiotics: rifampicin (50 μg ml −1 ), gentamycin (40 μg ml −1 ), tetracycline (5 µg ml −1 ) or kanamycin (25 μg ml −1 ) for A. tumefaciens , and rifampicin (20 µg ml −1 ), kanamycin (20 μg ml −1 ) or carbenicillin (50 μg ml −1 ) for A. rhizogenes . Plant materials and sterilisation Medicago sativa seeds were sterilised with 95% ethanol for 45 min followed by 6% sodium hypochlorite for 5 min, and germinated on distilled water agar in the dark for 2 days at room temperature. Pisium sativum seeds were sterilized with 70% ethanol for 1 min, washed with water, and then with 2% sodium hypochlorite for 5 min, rinsed thoroughly and germinated on distilled water agar in the dark for 2 days at room temperature. Medicago truncatula ecotype Jester was used for A. rhizogenes transformation. Seeds were scarified with sand paper, sterilised in 1% sodium hypochlorite for 3 min, incubated on agar (1.5%) in the dark for 3 days at 4 °C for stratification and then overnight at room temperature for germination. Seed sterilization and germination of spring barley genotype Golden Promise was performed using standard protocols [35] . Briefly, barley seeds were washed in 70% ethanol for 3 min, sterilised in 5% sodium hypochlorite for 4 min, incubated on agar (0.8%) in the dark for 3 days at 4 °C for stratification and then 3 days at room temperature for germination. Bacterial genetic manipulations and plasmid construction PCR was performed with Phusion High-Fidelity DNA Polymerase (Thermo Fisher Scientific) using primers in Supplementary Table 4 . 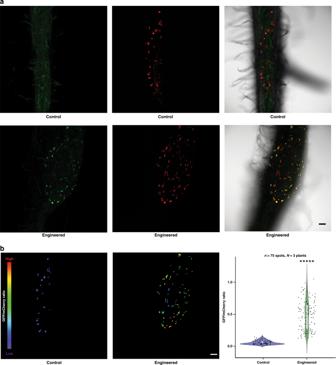Fig. 4 Fluorescent microscopy of rhizopine-mediated transkingdom signalling.aConfocal fluorescence microscopy images showing green fluorescent protein (GFP) fluorescence of Rlv3841::mTn7-mCherry/pOPS0761 biosensor [with constitutive mCherry fluorescence] on the surface of T1barley seedlings transformed with empty vector (control) or IdhA-MosB together (engineered). Z-stack projections of green fluorescence channel (left, GFP), red fluorescence channel (middle, mCherry) and all channels merged (right, bright-field) are shown (scale bars, 100 µm). Images shown are representative of experiments repeated two independent times.bThree-dimensional images of GFP/mCherry mean intensity ratios in Rlv3841::mTn7-mCherry/pOPS0761 biosensor on the surface of T1barley seedlings transformed with empty vector (left, control) or IdhA-MosB together (middle, engineered) (scale bars, 100 µm). Cool colours (purple) indicate low GFP/mCherry intensity ratio, and warm colours (red) indicate a high GFP/mCherry intensity ratio. Violin plot of GFP/mCherry ratios in the biosensor colonies (right;n> 75 spots;N= 3 plants). Asterisks signify statistical significance (Wilcoxon’s signed-rank test,P= 1.30 × 10−14). Images shown are representative of experiments repeated two independent times The biosensor pOPS0046 was constructed by restriction/ligation of a mocRB amplicon from S. meliloti L5-30 [36] into pIJ11268 [36] . Plasmids for pK19 mutant construction (pOPS0243, pOPS0244) were constructed by cloning internal fragments of S. meliloti L5-30 mosB and mosD into pK19mob [37] by BD In-Fusion cloning (Clontech). The plasmid for IolG purification (pOPS0241) was constructed by BD cloning of Bacillus subtilis iolG into pOPINF [38] . The plasmid for nodule expression of mosDEF (pOPS0362) was constructed using Saccharomyces cerevisiae homologous recombination [39] . A modified version of the Gram-negative expression vector pMQ131 [40] that contained the par locus for stability in the environment was used for recombineering with PmosB and mosDEF amplicons from S. meliloti L5-30. The plasmid pOPS0363 used for MosB purification was assembled by golden gate cloning [41] , [42] , [43] . Sinorhizobium meliloti tauR/Ptau taurine promoter, HIS-tagged maltose-binding protein, E. coli codon optimised mosB and rrnBT1 terminator were assembled in linear order into pOGG024 [44] . The rhizopine GFP biosensor plasmid pOPS0761 was constructed by assembly of the mocRB amplicon from pOPS0046 with an amplicon containing the GFPmut3 open reading frame into the modified pMQ131 vector described above by S. cerevisiae homologous recombination [39] . The resulting plasmid was conjugated into Rlv3841::mTn7-mCherry (Rlv3841 containing constitutively expressed mCherry introduced into the genome with pUC18T-miniTn7T-Gm [45] , [46] ). All plasmids were verified by restriction digest and DNA sequencing. 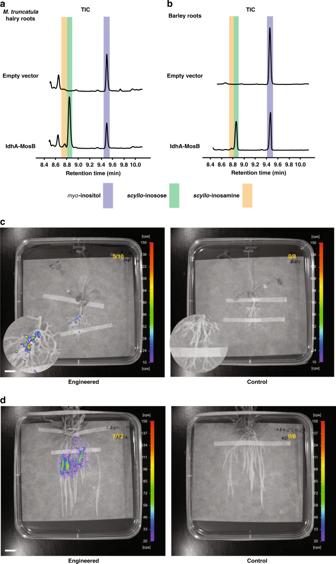Plasmids were transferred by conjugation into rhizobia by tri-parental mating with pRK2013 [47] . Fig. 3 Rhizopine biosynthesis and signalling inM. truncatulaand barley roots.a,bGas chromatography-mass spectrometry (GC-MS) total ion chromatograms (TICs) of extracts prepared fromM. truncatulatransgenic roots (a) and transgenic T0barley seedlings (b) transformed with empty vector (control) or IdhA-MosB together. Highlighted peaks indicatescyllo-inosamine1(orange),scyllo-inosose7(green) andmyo-inositol 3 (dark blue). All chromatograms are representative of experiments repeated at least three independent times. Source data for GC-MS chromatograms are provided as aSource Datafile in Supplementary Materials.c,dNightOwl images showing bioluminescence of Rlv3841/pOPS0046 rhizopineluxbiosensor on the surface ofM. truncatulatransgenic roots (c) and T0barley seedlings (d) transformed with empty vector (control) or IdhA-MosB together (engineered). Numbers in top right corners indicate number of plants tested that showed significant levels of bioluminescence (scale bar, 1 cm). Colours represent luminescence intensity from 10 or 20 counts per second (cool/purple) to 150 counts per second (warm/red). Source data underlyinga,bare provided as aSource Datafile Generation of constructs for plant engineering Constructs for plant engineering were assembled using golden gate cloning [41] , [42] , [43] (Supplementary Table 3 ). For transient expression, R. leguminosarum idhA and S. meliloti L5-30 mosB were expressed under the control of CaMV 35s promoter (35s) and Lotus japonicus Ubiquitin1 (LjUBI1) promoter, respectively. Sinorhizobium meliloti mosDEF and M. crystallinum IMT were expressed transiently under the control of 35s and LjUBI1 promoters, respectively. In barley transgenic lines, idhA and mosB were expressed under the control of Zea mays ubiquitin1 promoter and Oryza sativa ubiquitin1 promoter, respectively. All bacterial genes were codon optimised [48] for expression in plants. DNA components (promoters, coding sequences and terminators) were synthesised by GeneArt (Life Technologies). Recombinant clones were verified by PCR and DNA sequence analysis. Primers used are listed in Supplementary Table 4 . Bioinformatic identification of rhizopine loci Putative rhizopine loci were identified by BLAST query of the Joint Genome Institute Integrated Microbial Genomes (IMG) database ( https://img.jgi.doe.gov/ ) with S. meliloti L5-30 MosB and the IMG Ortholog Neighbourhood Viewer tool [49] . Putative rhizopine loci in other bacteria were selected that contained homologues to either mosC or mosA in addition to mosB . Genetic diagrams of the loci were copied from the IMG website and redrawn with Adobe Illustrator. Metabolite extraction and GC-MS analysis of root nodules Growth of M. sativa or P. sativum plants for nodule extraction was carried out in 1 L pots filled with sterile vermiculite and nitrogen (N 2 )-free rooting solution [50] . Ten germinated M. sativa or two germinated P. sativum seedlings per pot were inoculated with 1 × 10 7 colony-forming units (CFUs) of rhizobia in distilled water 3 days after planting. Plants were grown for 6 to 8 weeks before harvesting pink N 2 -fixing nodules by hand. Pooled nodules from one pot (<100 mg) were ground using a mortar and pestle in liquid nitrogen. Enzymes were inactivated by the addition of 1400 μl 100% methanol and incubated for 10 min at 70 °C. For metabolite extraction, 750 μl of CHCl 3 and 1400 μl of dH 2 O was added, samples were vortexed and then centrifuged for 15 min at a relative centrifugal force (RCF) of 2200. Aliquots of the supernatant were then dried in a vacuum concentrator prior to derivitization [51] . Samples were derivatised by trimethylsilylation prior to GC-MS analysis by incubation with 25 μl of pyridine and 35 μl of trimethylsilylimidazole (TMSI) (Sigma 33068) for 60 min at 37 °C with shaking at 950 RPM. GC-MS analysis was performed using the LJS_TMSI protocol at the University of Oxford Department of Plant Sciences (Supplementary Methods). For data generated in Supplementary Fig. 5 , GC-MS was performed with the LJS_Golm Stardard protocol (Supplementary Methods). Protein purification For purification of IolG and IdhA, pOPS0141 and pOPS0142 were transformed into BL21-competent E. coli (New England Biolabs) and grown overnight in 5 ml LB Amp . The next day, the full volume was subcultured to 50 ml LB Amp . At OD 600 (optical density at 600 nm) of 0.5, 1 mM isopropyl β- d -1-thiogalactopyranoside (IPTG) was added. After 3 h of induction cells were pelleted at 4 °C, frozen with liquid nitrogen and stored at −80 °C. Cell pellets were thawed on ice, resuspended in 1 ml of HIS-binding buffer and disrupted by ribolyzing. Lysate was clarified by centrifugation at 4 °C. Purification of HIS-tagged proteins from the lysate was performed using a His-Spin Protein Miniprep Kit (Zymo Research). For purification of MosB, R. leguminosarum 3841 maintaining pOPS0363 was grown on a TY agar slope with antibiotics for 3 days, washed with UMS and used to inoculate six baffled flasks containing 500 ml of UMS (containing 20 mM succinate, 10 mM NH 4 Cl and 10 mM taurine) to OD 600 of 0.01. Cultures were grown until they reached an OD 600 of 0.5, pelleted at 4 °C, frozen in liquid nitrogen and stored at −80 °C. Cell pellets were thawed on ice and resuspended in 15 ml extraction buffer (MBPTrap binding buffer (20 mM Tris-HCl, 200 mM NaCl, 1 mM EDTA, pH 7.4) containing 1 mM dithiothreitol and PMSF Protease Inhibitor (Thermo Fisher)). Cells were disrupted by ribolysing and clarified by centrifugation at 4 °C. The clarified lysate was filtered (0.45 μm) and loaded onto a 1 ml MBPTrap HP column on an AKTA Basic 10 (GE Healthcare Life Sciences). The column was washed with running buffer and eluted with running buffer containing 10 mM maltose. Purity of purified proteins was assessed by sodium dodecyl sulfate-polyacrylamide gel electrophoresis analysis and proteins were quantified using a Qubit 2.0 Fluorometer (Thermo Fisher) according to the manufacturer’s instructions. MosB in vitro assays The MosB in vitro assay contained 100 mM Tris-HCl, pH 7.5, 0.9 mM PLP, 5 mM (±)-3- O -methyl- scyllo -inosose (±)- 6 and 5 mM of amino acid and water to a total volume of 100 μl (±)-3- O -methyl- scyllo -inosose (±)- 6 was used immediately following its synthesis due to instabilities observed. The linked assay with IolG used the reaction mixture described above, as well as 5 mM NAD + and 5 mM myo- inositol 3 as substrate rather than 3- O -methyl- scyllo -inosose. Proteins were added to a concentration of 10 μg ml −1 . Assays were incubated for 24 h at 28 °C. Enzyme activity was halted by boiling for 10 min and protein was removed by centrifugation. The supernatant was dried in a vacuum centrifuge and derivatised by resuspending in 25 μl pyridine and 35 μl TMSI at 37 °C with shaking for 60 min. GC-MS analysis was performed with the LJS_TMSI protocol at the University of Oxford Department of Plant Sciences (Supplementary Methods). Transient expression in Nicotiana benthamiana Recombinant plasmids were mobilised into A. tumefaciens GV3101:pMP90 by electroporation. A transformed single colony was grown in LB with appropriate antibiotics for 24 h, and then subcultured in fresh LB and grown overnight. Cells were harvested by centrifugation and resuspended in infiltration buffer (10 mM MES buffer, pH 5.6, 10 mM MgCl 2 and 150 µM acetosyringone) to an OD 600 of 0.5. After incubating at room temperature in the dark for 3 h, A. tumefaciens strains were mixed with an equal volume of a P19 suppressor strain and infiltrated into the underside of N. benthamiana leaves using a needleless 1 ml syringe. Leaf discs were harvested 3 days after infiltration, frozen in liquid nitrogen and the extracted metabolites were analysed by GC-MS. Hairy-root transformation in Medicago truncatula Agrobacterium rhizogenes AR1193 was transformed with recombinant constructs by electroporation. A transformed single colony was grown on LB agar plates with antibiotics for 48 h. Cells were removed using sterile toothpicks and suspended in 1 ml of sterile water. Germinated seedlings of M. truncatula cultivar Jester were transformed with A. rhizogenes AR1193 using standard protocols [52] . Briefly, under sterile conditions cut tip of radicle approximately 3 mm from the root tip of each germinated seedlings, dip the ends of each cut seedlings into A. rhizogenes AR1193 culture and grown them on ModFP agar plates. Four weeks after transformation, composite plants were screened on the basis of fluorescent enhanced GRP (eGFP) marker. eGFP-positive transgenic roots were harvested and frozen in liquid nitrogen before extracting metabolites for GC-MS analysis. For cultivation of axenic hairy-root cultures, 4 weeks after transformation of M. truncatula seedlings by A. rhizogenes AR1193, transgenic roots of approximately 3 to 5 cm in length were excised and subcultured every 3 weeks on M agar plates containing 350 µg ml −1 of cefotaxime sodium. For GC-MS analysis, 3-week-old transgenic hairy-root organ cultures grown on Modified M agar plates (containing 0.4 mM NH 4 NO 3 ) were harvested, frozen in liquid nitrogen and extracted metabolites were analysed. Stable transformation of Hordeum vulgare Recombinant binary vectors were transferred by electroporation into A. tumefaciens AGL1 strain. Transformation of barley by recombinant Agrobacterium strains was performed using standard protocols [35] . For rapid testing in T 0 barley plants, approximately 12 weeks after transformation, transgenic roots from barley plantlets were harvested, frozen in liquid nitrogen and the extracted metabolites were analysed by GC-MS. Approximately 2-week-old T 1 barley plants were used for confocal microscopy and GC-MS analysis. GC-MS analysis of engineered plant tissue Frozen plant materials were lyophilized to dryness, ground to a fine powder and extracted with 70% ethanol at 70 °C for 60 min. The resulting extract was centrifuged at an RCF of 15,871 or 10 min and the supernatant was evaporated to dryness. For GC-MS analysis, dried metabolic samples were dissolved in appropriate volume of 70% ethanol, 50 μl aliquots were dried down and trimethylsilylated using Tri-Sil Z reagent (Sigma, catalogue no. 92718) at 80 °C for 60 min. GC-MS analysis was performed using the Eng_Plant protocol at the John Innes Centre (Supplementary Methods). Rhizopine production in engineered plant samples were determined using a calibration curve (concentration vs. peak area) drawn by analysing a set of rhizopine standards of known concentrations in GC-MS. MassHunter qualitative analysis software (Agilent) was used to determine the peak area of rhizopine in EIC ( m / z 245) chromatograms of the standards and plant samples. Bacterial luciferase biosensor screening assays For imaging of rhizopine synthesis in M. sativa sterilised, germinated seedlings were placed onto square plates containing FP-agar overlaid with filter paper. Roots were inoculated at the time of planting with 5 × 10 7 cells ( S. meliloti L5-30 strain and R. leguminosarum Rlv3841 carrying the rhizopine lux biosensor mixed 1:1) [20] . Plants were imaged after the formation of N 2 -fixing nodules at 2 weeks post inoculation. For imaging rhizopine secretion on transgenic M. truncatula hairy roots, 4-week-old composite plants with transgenic roots were transferred to new ModFP agar plates and inoculated with Rlv3841 carrying the rhizopine lux biosensor. For transgenic M. truncatula root organ cultures, 1-week-old hairy-root explants were transferred to new Modified M agar plates without antibiotics and inoculated with R. leguminosarum Rlv3841 carrying the rhizopine lux biosensor. Both transgenic M. truncatula hairy roots and root organ cultures were imaged every week post inoculation. For imaging rhizopines secretion on transgenic T 0 barley plant roots, approximately 12-week-old primary T 0 barley transformants with strong root growth were transferred from regeneration medium to ModFP agar petridishes without antibiotics and R. leguminosarum Rlv3841 carrying the rhizopine lux biosensor was inoculated on the engineered roots. Plants were imaged each day post-inoculation. Bioluminescence images were analysed for quantification using imaging software IndiGO (Berthold Technologies) and data were expressed as the ratio of luminescence to surface (cps mm −2 ). Confocal microscopy and image analysis For imaging rhizopine-mediated signalling on transgenic T 1 barley plant roots, 3-day-old germinated seedlings were grown in ModFP agar Petri dishes and Rlv3841 strain carrying the rhizopine GFP-mCherry biosensor was inoculated on the engineered roots. Plants were imaged from 10 days post inoculation. Confocal images were taken using a Leica SP8-FLIMan with an HC PLAN APO ×10/0.40 dry objective. The 488 and 552 nm lasers were used to excite GFP and red fluorescent protein (mCherry), respectively. Fluorescence emissions were collected using HyD SMD detectors set to detect GFP (500–530 nm) and mCherry (600–630 nm). The 488 and 552 nm lasers were set at 4 and 2% with detector gain at 12 and 36 for GFP and mCherry protein fluorescence imaging, respectively. A line average of three was used and z-slices were acquired with a step size of 2.41 µm. Confocal images were analysed using IMARIS 8.3.1 (Bitplane) and ImageJ software’s. Image processing and analysis were done using IMARIS 8.3.1 as previously described [53] . Briefly, mCherry (RFP) channel was used to segment surfaces (i.e. individual bacterial colonies) using the ‘surfaces wizard’ with background subtraction and thresholding set at default values 11 µm and 361, respectively. Surfaces were false-coloured based on the mean of the masked GFP and mCherry (RFP) channels. IMARIS Xtension ‘XT Mean Intensity Ratio’ was used to calculate the GFP/mCherry intensity ratio of individual surfaces [53] . The mean intensity ratios (GFP/mCherry) was presented in a violin plot drawn by using R-programming. Wilcoxon’s signed-rank test analysis was used to test the level of significance. Analysis of growth and bioreporter expression in culture Analysis of expression of bioreporters in free-living culture was performed with either a FLUOstar OMEGA (Lite) or CLARIOstar plate reader (BMG Labtech). Strains were grown in UMS-defined medium with a starting OD 600 of 0.1. UMS was supplemented with either 30 mM sodium pyruvate as a carbon source or 10 mM NH 4 Cl as a nitrogen source. Cultures were grown and monitored in black 24-well plates clear bottom plates covered with a gas-permeable moisture barrier seal (4titude) at 28 °C shaking at 500 RPM on the orbital setting. Measurements of luminescence were taken at 30-min intervals. Data are expressed as relative luminescence units calculated from total luminescence per well/ culture density measured by OD 595 . Reporting summary Further information on research design is available in the Nature Research Reporting Summary linked to this article.